An ITAM-Syk-CARD9 signalling axis triggers contact hypersensitivity by stimulating IL-1 production in dendritic cells A variety of reactive organic compounds, called haptens, can cause allergic contact dermatitis. However, the innate immune mechanisms by which haptens stimulate dendritic cells (DCs) to sensitize T cells remain unclear. Here we show that the coupling of ITAM-Syk-CARD9 signalling to interleukin-1 (IL-1) secretion in DCs is crucial for allergic sensitization to haptens. Both MyD88 and Caspase recruitment domain-containing protein 9 (CARD9) signalling are required for contact hypersensitivity (CHS). Naïve T cells require signals received through IL-1R1-MyD88 for effector differentiation, whereas DCs require CARD9 and spleen tyrosine kinase (Syk) signalling for hapten-induced IL-1α/β secretion and their ability to prime T cells. DC-specific deletion of CARD9, DAP12, Syk or NLRP3, but not MyD88, is sufficient to abolish CHS. All tested haptens, but not irritants, can induce Syk activation, leading to both the CARD9/BCL10-dependent pro-IL-1 synthesis (signal1) and reactive oxygen species-mediated NLRP3 inflammasome activation (signal2), required for IL-1 secretion. These data unveil an innate immune mechanism crucial for allergic contact sensitization to chemical compounds. Allergic contact dermatitis (ACD) is caused by the reaction of T cells to various environmental and industrial allergens, including inorganic metals such as nickel and cobalt, and various small reactive organic compounds called haptens [1] . Over 2,800 chemical compounds have been identified to have the potential to cause ACD. Haptens can penetrate the skin upon contact and bind to proteins to form hapten self-protein complexes, which are recognized by the immune system as an ‘altered-self’ antigen. Skin-resident dendritic cells (DCs), such as Langerhans cells and dermal DCs, capture the haptenated proteins and migrate to the skin-draining lymph nodes (dLNs), where they prime hapten-specific T cells, a process called ‘sensitization’. Re-exposure to haptens elicits accumulation of effector T cells in the skin, where they release pro-inflammatory cytokines and destroy haptenated cells through cytotoxic activity [2] , [3] , resulting in the development of eczema. Hapten-specific CD8 T cells producing interleukin-17 (IL-17) and IFNγ (Tc1 and Tc17) are the primary effector T cells that mediate the elicitation response [4] , [5] . It has long been recognized that the triggering of T-cell receptors (TCRs) by peptide–MHC complex alone is insufficient to prime naïve T cells to drive effector T-cell differentiation. Additional signals, including co-stimulatory signals and cytokines, delivered by activated antigen-presenting DCs are also required. DC activation depends on activation of the innate immune system through pattern-recognition receptors that sense microbial or endogenous danger products [6] , [7] , [8] . Toll-like receptor (TLR) 4 in humans was shown to play a crucial role for the development of contact allergy to nickel and cobalt by directly binding to them and inducing pro-inflammatory gene expression [9] , [10] . However, the innate immune mechanisms by which structurally varied haptens are sensed by and activate skin DCs are uncertain. A previous report described the involvement of TLR2 and TLR4 for the induction of contact hypersensitivity (CHS) by haptens [11] . TLR2/4 may be activated by breakdown products of hyaluronic acid, a component of the extracellular matrix [12] , generated by reactive oxygen species (ROS) induced by haptens [12] , [13] , [14] . However, DCs primed in vitro with haptens in the absence of hyaluronic acid are capable of sensitizing CHS [11] , [15] . In addition, myeloid differentiation primary response 88 (MyD88), an essential signalling adaptor protein mediating signalling by most TLRs and IL-1 family receptors, was dispensable in LCs for CHS [16] . These results suggest the presence of alternative innate immune pathways that activate skin DCs so that they can prime hapten-specific T cells. IL-1α and IL-1β are involved in the pathogenesis of various inflammatory disorders [17] , [18] and they both mediate their biological activities via IL-1 receptor type I (IL-1R1). It is well documented that the secretion of biologically active IL-1β is regulated by two signals: first, increased transcription of the IL-1β gene and production of cytosolic pro-IL-1β (signal 1), which are dependent on the activation of NF-κB via pattern-recognition receptors; and second, autoproteolytic activation of caspase-1 (signal 2), which cleaves pro-IL-1β and allows secretion of mature IL-1β, mediated by cytoplasmic multiprotein complexes called inflammasomes that sense pathogen-associated molecular patterns and endogenous danger-associated molecules [19] . The NLRP3 inflammasome is the best characterized inflammasome and is engaged by structurally and chemically diverse stimuli [20] . Previous reports suggested that IL-1α, IL-1β and IL-1R1 signalling were crucial for the development of CHS in a mouse model of ACD [21] , [22] , [23] , [24] , [25] , [26] . In addition, it has been reported that mice lacking the NLRP3 inflammasome components, NLRP3 or ASC, are resistant to CHS [15] , [27] . Watanabe et al . [27] reported that ASC deficiency resulted in impaired Caspase-1 activation in response to haptens in keratinocytes. Furthermore, Weber et al . [15] reported that the capacity to initiate CHS was impaired in DCs from NLRP3 or ASC knockout mice. Thus, NLRP3 inflammasome-dependent IL-1 production is important for the development of CHS. However, the molecular and cellular networks by which IL-1 acts to trigger CHS remain unclear. In addition, although the ATP receptor P2X 7 has been suggested to be involved in CHS [15] , the mechanisms that sense haptens and trigger signals for inflammasome activation are also yet to be defined. Caspase recruitment domain-containing protein 9 (CARD9) forms a complex with B-cell lymphoma 10 (BCL10) and functions as an essential signalling adaptor protein in nuclear factor-κB (NF-κB) signalling through immunoreceptor tyrosine-based activation motifs (ITAM)-coupled receptors in myeloid cells [28] , such as C-type lectin receptors (CLRs), CD300/LMIR family receptors and TREM family receptors [29] , [30] , [31] . Most of these receptors signal through the spleen tyrosine kinase (Syk) by association with the ITAM-containing adaptors, that is, DNAX-activating protein of 12 kDa (DAP12) or FcRγ chain. Syk-CARD9-dependent signals through CLRs, such as Dectin-1, -2 and Mincle, play a critical role in the innate immune response to fungi and the antifungal defence by regulating protective Th17 development [32] , [33] , [34] . In this study, we show that the coupling of ITAM-Syk-CARD9/BCL10 signalling to the NLRP3 inflammasome in DCs plays a crucial role for allergic sensitization to haptens. Stimulation of DCs in vitro with haptens, but not irritants, induces both IL-1α and IL-1β secretion in a manner dependent on NLRP3, ITAM-Syk and CARD9, but not Myd88, signalling. The hapten-induced IL-1 secretion by DCs is required for their ability to prime T cells, while receiving signals through IL-1R1-MyD88 upon priming is required for naïve T cells to differentiate into effectors, both in vitro and in vivo . ITAM-Syk signalling controls both pro-IL-1 synthesis (signal 1) and triggering of NLRP3 inflammasome (signal 2) after hapten stimulation. On the other hand, CARD9/Bcl10 selectively controls signal 1 by regulating NF-κB activation. Thus, our data reveal an innate signalling axis essential for allergic sensitization to haptens and unveil an important immunological property of haptens likely associated with their allergenicity. CARD9 in DCs is required for hapten sensitization CARD9 and MyD88 are important signalling adaptors involved in innate immune activation of antigen-presenting cells. To explore the innate immune pathways involved in CHS, we tested the impact of MyD88 or CARD9 deficiency on the development of CHS to a hapten, 2,4,6-trinitro-1-chlorobenzene (TNCB). We found that both MyD88 −/− and CARD9 −/− mice failed to develop CHS characterized by oedema (swelling) ( Fig. 1a ) and mononuclear cell infiltration ( Fig. 1b ) in the skin. In contrast, neither deficiency affected the development of irritant dermatitis induced by the application of sodium lauryl sulphate (SLS) ( Fig. 1c ). Ex vivo analyses of hapten-specific IFN-γ and IL-17A production by T cells isolated from skin dLNs (dLNs) of the sensitized mice revealed that effector T-cell differentiation was markedly impaired in both MyD88 −/− and CARD9 −/− mice ( Fig. 1d ). In addition, dLN T cells from TNCB-sensitized MyD88 −/− or CARD9 −/− mice could not adoptively transfer CHS to naïve WT recipient mice, whereas those from sensitized WT mice transferred CHS to naïve WT, MyD88 −/− and CARD9 −/− recipient mice ( Supplementary Fig.1a,b ). These data suggest that both MyD88- and CARD9-mediated signals are required for the sensitization of hapten-specific T cells, but are dispensable for the CHS reaction elicited by sensitized T cells. 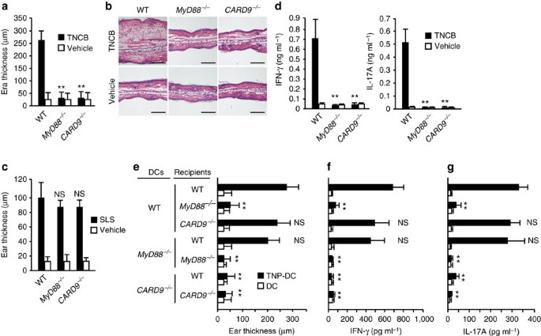Figure 1: Both CARD9 and MyD88 signalling are indispensable for the sensitization to contact allergens. (a) WT,MyD88−/−andCARD9−/−mice (n=5 per group) were sensitized with TNCB or acetone (vehicle). On day 5 after sensitization, ear swelling at 24 h after challenge with TNCB were measured (means±s.d.,**P<0.01 by Student’st-test). (b) Histology (H&E staining) inaafter challenge. Data are representative of three independent experiments. Scale bars, 200 μm. (c) Irritant dermatitis. SLS or DMF (vehicle) was applied to the ear skin of WT,MyD88−/−andCARD9−/−mice and ear swelling at 24 h was measured (means±s.d.;n=5 per group; NS, not significant by Student’st-test). (d) Skin dLN T cells were isolated from TNCB-sensitized mice inaand stimulatedin vitrofor 3 days with irradiated syngeneic spleen cells pretreated with TNBS. IFN-γ and IL-17A production in the culture was measured by ELISA (means±s.d.,n=5 per group;**P<0.01 by Student’st-test). (e) CHS induction by TNP-modified BMDCs. WT,MyD88−/−orCARD9−/−mice were intracutaneously injected with 3 × 105of TNP-modified (TNP-DC) or unmodified (DC) WT,MyD88−/−orCARD9−/−BMDCs. Five days after the injection, ear swelling 24 h after TNCB challenge was measured (means±s.d.,n=5 per group,**P<0.01 by Student’st-test). (f,g) T cells from skin dLNs of the sensitized mice inewere stimulated with irradiated syngeneic spleen cells modified with TNP and the production of IFN-γ (f) and IL-17A (g) was measured by ELISA (means±s.d.,n=5 per group;**P<0.01 by Student’st-test). Figure 1: Both CARD9 and MyD88 signalling are indispensable for the sensitization to contact allergens. ( a ) WT, MyD88 −/− and CARD9 −/− mice ( n =5 per group) were sensitized with TNCB or acetone (vehicle). On day 5 after sensitization, ear swelling at 24 h after challenge with TNCB were measured (means±s.d., **P <0.01 by Student’s t- test). ( b ) Histology (H&E staining) in a after challenge. Data are representative of three independent experiments. Scale bars, 200 μm. ( c ) Irritant dermatitis. SLS or DMF (vehicle) was applied to the ear skin of WT, MyD88 −/− and CARD9 −/− mice and ear swelling at 24 h was measured (means±s.d. ; n =5 per group; NS, not significant by Student’s t- test). ( d ) Skin dLN T cells were isolated from TNCB-sensitized mice in a and stimulated in vitro for 3 days with irradiated syngeneic spleen cells pretreated with TNBS. IFN-γ and IL-17A production in the culture was measured by ELISA (means±s.d., n =5 per group; **P< 0.01 by Student’s t- test). ( e ) CHS induction by TNP-modified BMDCs. WT, MyD88 −/− or CARD9 −/− mice were intracutaneously injected with 3 × 10 5 of TNP-modified (TNP-DC) or unmodified (DC) WT, MyD88 −/− or CARD9 −/− BMDCs. Five days after the injection, ear swelling 24 h after TNCB challenge was measured (means±s.d., n =5 per group, **P <0.01 by Student’s t- test). ( f , g ) T cells from skin dLNs of the sensitized mice in e were stimulated with irradiated syngeneic spleen cells modified with TNP and the production of IFN-γ ( f ) and IL-17A ( g ) was measured by ELISA (means±s.d., n =5 per group; **P <0.01 by Student’s t- test). Full size image To examine whether MyD88 or CARD9 deficiency affects the ability of DCs to induce CHS, we sensitized mice by intracutaneous injection of TNP-modified, bone marrow-derived DCs (TNP-DCs) [35] from WT, MyD88 −/− or CARD9 −/− mice, and 5 days later, CHS reaction was examined. WT mice injected with WT or MyD88 −/− TNP-DCs developed a CHS response with ear swelling and inflammation after challenge, whereas mice injected with CARD9 −/− TNP-DCs failed to develop these responses ( Fig. 1e and Supplementary Fig. 2 ) because of defective generation of hapten-specific effector T cells ( Fig. 1f,g ) in the dLNs. These data suggest that signalling through CARD9 but not MyD88 is required for DCs to prime hapten-specific T cells. IL-1R1-MyD88 signal in T cells is required for hapten sensitization Interestingly, whereas loss of CARD9 in recipients did not affect disease severity, loss of MyD88 in recipients impaired CHS responses ( Fig. 1e ) and development of effector T cells in the skin dLNs ( Fig. 1f,g ). These data suggest that MyD88 signalling plays an essential role in non-DC recipient cells, albeit it is dispensable in DCs, for the sensitization of CHS. CHS is impaired in mice deficient in IL-1α, IL-1β or IL-1 receptor 1 (IL-1R1) [21] , [22] , [24] , [25] , [26] , [27] . In addition, IL-1 is a critical factor in the in vivo differentiation of IL-17-producing T cells [36] , [37] , [38] , which play pivotal roles in CHS reaction [4] . Because MyD88 mediates signals through the IL-1 and IL-18 receptors, we reasoned that signalling through IL-1R1 in T cells might be responsible for the defective CHS sensitization in MyD88 −/− mice. To examine it, first, we constructed an in vitro T-cell differentiation system by co-culturing naïve T cells with TNP-DCs in the presence of anti-CD3ε antibody. After 4 days of culture, effector T-cell differentiation was evaluated by measuring the production of IL-17A and IFN-γ after re-stimulation with phorbol myristate acetage (PMA) plus calcium ionophore. Differentiation of IL-17-producing T cells was substantially induced when DCs were stimulated with TNP or with stimulants that are known to induce IL-1 secretion, that is, lipopolysaccharide (LPS) plus adenosine triphosphate (ATP) (LPS+ATP) or the Dectin-1 agonist ox-zymosan ( Fig. 2a ). In contrast, although differentiation of IFN-γ-producing T cells was promoted by stimulation of DCs with LPS+ATP, which was strictly dependent on MyD88, it was not promoted by stimulation with TNP or ox-zymosan ( Supplementary Fig. 3 ). Intracellular staining revealed that the IL-17-producing T cells generated by TNP-modified WT DCs were mainly CD8 + cells, namely Tc17 cells ( Fig. 2b ). Consistent with the data in Fig. 1e , the Tc17 differentiation mediated by TNP-DCs required CARD9 but not MyD88 expression in DCs ( Fig. 2a ). Addition of IL-1 receptor antagonist to the culture attenuated the Tc17 differentiation induced by WT or MyD88 −/− TNP-DCs. In contrast, recombinant IL-1β restored Tc17 development in the CARD9 −/− TNP-DC culture. Moreover, Tc17 differentiation was completely abolished when MyD88 −/− or IL-1R1 −/− T cells were used for the culture. Collectively, these results suggest that IL-1R1-MyD88 signalling in T cells is essential for the differentiation of IL-17-producing effector T cells driven by TNP-activated DCs in vitro . 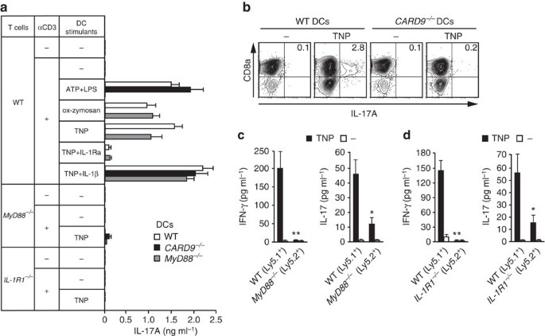Figure 2: T cells require MyD88 signalling through IL-1R1 for differentiation into effectors. (a,b)In vitroT-cell differentiation. Purified naïve LN T cells from WT,MyD88−/−orIL-1R1−/−mice were cultured with unmodified or TNP-modified BMDCs, or BMDCs stimulated with LPS+ATP or ox-zymosan, in the presence or absence of anti-CD3ε mAb (1 μg ml−1) with or without recombinant IL-1β and IL-1 receptor antagonist. After 4 days of culture, T cells were re-stimulated with PMA (50 ng ml−1) plus a calcium ionophore (1 μM). (a) The secretion of IL-17A in the culture supernatant was measured using ELISA (means±s.d.,n=5 per group;**P<0.01 by Student’st-test). (b) Flow cytometric analysis of intracellular IL-17A expression in WT T cells that were differentiated with unmodified or TNP-modified WT orCARD9−/−BMDCs in the presence of anti-CD3ε mAb. Percentages of CD8α+IL-17A-positive cells are shown. (c,d)Rag2−/−mice (n=3 per group) were reconstituted with naive T cells from WT (Ly5.1+) mice andMyD88−/−(Ly5.2+) mice (c), or from WT (Ly5.1+) andIL-1R1−/−(Ly5.2+) mice (d). Then, mice were epicutaneously sensitized to TNCB and 5 days later, skin dLN cells were collected and sorted into Ly5.1+and Ly5.2+T cells using a FACS cell sorter. The T cells were cultured for 3 days with irradiated syngeneic spleen cells modified (black bars) or unmodified (white bars) with TNP. IFN-γ and IL-17A production in the culture supernatant was measured by ELISA (means±s.d.,n=3 per group;*P<0.05 and**P<0.01 by Student’st-test). Figure 2: T cells require MyD88 signalling through IL-1R1 for differentiation into effectors. ( a , b ) In vitro T-cell differentiation. Purified naïve LN T cells from WT, MyD88 −/− or IL-1R1 −/− mice were cultured with unmodified or TNP-modified BMDCs, or BMDCs stimulated with LPS+ATP or ox-zymosan, in the presence or absence of anti-CD3ε mAb (1 μg ml −1 ) with or without recombinant IL-1β and IL-1 receptor antagonist. After 4 days of culture, T cells were re-stimulated with PMA (50 ng ml −1 ) plus a calcium ionophore (1 μM). ( a ) The secretion of IL-17A in the culture supernatant was measured using ELISA (means±s.d., n =5 per group; **P <0.01 by Student’s t- test). ( b ) Flow cytometric analysis of intracellular IL-17A expression in WT T cells that were differentiated with unmodified or TNP-modified WT or CARD9 −/− BMDCs in the presence of anti-CD3ε mAb. Percentages of CD8α + IL-17A-positive cells are shown. ( c , d ) Rag2 −/− mice ( n =3 per group) were reconstituted with naive T cells from WT (Ly5.1 + ) mice and MyD88 −/− (Ly5.2 + ) mice ( c ), or from WT (Ly5.1 + ) and IL-1R1 −/− (Ly5.2 + ) mice ( d ). Then, mice were epicutaneously sensitized to TNCB and 5 days later, skin dLN cells were collected and sorted into Ly5.1 + and Ly5.2 + T cells using a FACS cell sorter. The T cells were cultured for 3 days with irradiated syngeneic spleen cells modified (black bars) or unmodified (white bars) with TNP. IFN-γ and IL-17A production in the culture supernatant was measured by ELISA (means±s.d., n =3 per group; *P <0.05 and **P< 0.01 by Student’s t- test). Full size image Next, we sought to determine the importance of IL-1R-MyD88 signalling for T-cell priming in vivo . To compare the ability of WT and IL-1R1 −/− or MyD88 −/− T cells to differentiate into effector T cells under the same in vivo conditions, we reconstituted T cell-deficient Rag2 −/− mice with a 1:1 mixture of naïve T cells from Ly5.1 congenic WT mice and Ly5.2 congenic IL-1R1 −/− or MyD88 −/− mice, and then, we epicutaneously sensitized mice with TNCB. Five days later, skin dLN cells were collected and sorted into Ly5.1 + (WT) and Ly5.2 + ( IL-1R1 −/− or MyD88 −/− ) T cells and compared cytokine response with the hapten. Production of IL-17 and IFN-γ in response to TNP was markedly reduced in MyD88 −/− ( Fig. 2c ) or IL-1R1 −/− ( Fig. 2d ) T cells relative to WT T cells. Thus, these data indicate that IL-1R1-MyD88 signalling in T cells is crucial for differentiation of both IL-17- and IFN-γ− producing effector T cells in vivo during sensitization for CHS. DAP12-CARD9 signal controls hapten-induced IL-1 secretion Our data so far indicate that haptens could directly induce IL-1 production by DCs, and which is important for priming of hapten-specific T cells in dLNs. We found that trinitrobenzene sulphonic acid (TNBS) stimulation in vitro induced both IL-1α and IL-1β secretion by BMDCs ( Fig. 3a ). Because it has been reported that caspase-1 activation regulated by the NLRP3 inflammasome is involved in the CHS response [15] , we examined whether the NLRP3 inflammasome is required for hapten-induced IL-1α/β production. Both IL-1α and IL-1β production after TNBS stimulation was dependent on NLRP3 as well as caspase-1 ( Fig. 3a ). In line with the ability to sensitize CHS, CARD9 −/− but not MyD88 −/− DCs failed to produce both IL-1α and IL-1β in response to TNBS, whereas loss of CARD9 did not influence their production after stimulation with other NLRP3 inflammasome activators, LPS+ATP or silica, or with the AIM2 inflammasome activator, double-stranded DNA (poly (dA:dT)) ( Fig. 3a,b ). As CARD9 mediates signal activation through myeloid ITAM-coupled receptors [28] , we next tested whether the ITAM-containing adaptors DAP12 and FcRγ are involved in the hapten-induced IL-1 production. We found that DAP12 −/− DCs failed to produce both IL-1α and IL-1β after TNBS stimulation as CARD9 −/− DCs, whereas loss of FcRγ did not affect the IL-1α/β production ( Fig. 3c ). DAP12 deficiency did not affect IL-1α/β production after stimulation not only with LPS+ATP or poly (dA:dT) but also with ox-zymosan, a Dectin-1 ligand that induces IL-1α/β secretion in a CARD9-dependent fashion. Therefore, DAP12 specifically controls the signalling pathway that couples hapten stimulation to IL-1α/β secretion upstream of CARD9. In addition, similarly to CARD9 deficiency, loss of DAP12 or NLRP3, but not FcRγ, abrogated the ability of TNP-DCs to sensitize CHS ( Fig. 3d–f and Supplementary Fig. 4 ). 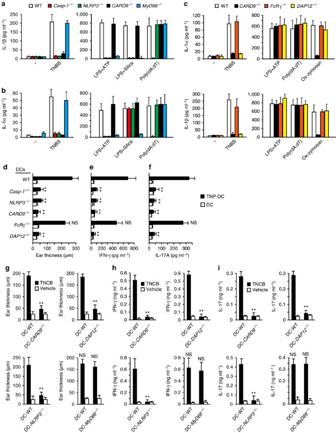Figure 3: DAP12-CARD9 signalling and NLRP3 are essential for contact allergen-induced IL-1α/β secretion and the capacity of DCs to induce CHS. IL-1β (a) and IL-1α (b) secretion by BMDCs from indicated mice after stimulation with TNBS (100 μg ml−1), ATP (5 mM), silica (100 μg ml−1) or ox-zymosan (100 μg ml−1), or after transfection of poly (dA:dT) (2 μg ml−1) for 12 h. For ATP and silica stimulation, cells were primed with LPS (1 ng ml−1) for 3 h before stimulation (means±s.d.,n=3 per group). (c) IL-1α and -1β secretion by WT,CARD9−/−,FcRγ−/−andDAP12−/−BMDCs after stimulation as in a (means±s.d.,n=3 per group). (d–f) WT naïve mice were sensitized by intracutaneous injection of unmodified (DC) or TNP-modified BMDCs (TNP-DC) from indicated mice. After 5 days, ear-swelling responses after challenge (d) as well as TNP-specific IFN-γ (e) and IL-17A (f) production by skin dLN T cells were analysed (means±s.d.,n=5 per group,**P<0.01 by Student’st-test). (g) CHS in mice carrying DC-specific deletion of CARD9 (DC-CARD9−/−), DAP12 (DC-DAP12−/−), NLRP3 (DC-NLRP3−/−) or MyD88 (DC-MyD88−/−) generated by a method indicated inSupplementary Fig. 5. Chimeric mice were treated twice with DT 1 week apart and were sensitized with TNCB or vehicle on the abdominal skin. On day 5 after sensitization, ear swelling 24 h after challenge was analysed (means±s.d.,n=5 per group,**P<0.01 by Student’st-test). Data are representative of two independent experiments. (h,i) Hapten-specific cytokine response of dLN T cells isolated from DC-CARD9−/−, DC-DAP12−/−, DC-NLRP3−/−, DC-MyD88−/−and their respective control (DC-WT) mice 5 days after epicutaneous sensitization ing. T cells were stimulatedin vitrofor 3 days with irradiated spleen cells modified with TNP. IFN-γ (h) and IL-17A (i) production in the culture was measured by ELISA (means±s.d.,n=5 per group,**P<0.01 by Student’st-test). Figure 3: DAP12-CARD9 signalling and NLRP3 are essential for contact allergen-induced IL-1α/β secretion and the capacity of DCs to induce CHS. IL-1β ( a ) and IL-1α ( b ) secretion by BMDCs from indicated mice after stimulation with TNBS (100 μg ml −1 ), ATP (5 mM), silica (100 μg ml −1 ) or ox-zymosan (100 μg ml −1 ), or after transfection of poly (dA:dT) (2 μg ml −1 ) for 12 h. For ATP and silica stimulation, cells were primed with LPS (1 ng ml −1 ) for 3 h before stimulation (means±s.d., n =3 per group). ( c ) IL-1α and -1β secretion by WT, CARD9 −/− , FcRγ −/− and DAP12 −/− BMDCs after stimulation as in a (means±s.d., n =3 per group). ( d – f ) WT naïve mice were sensitized by intracutaneous injection of unmodified (DC) or TNP-modified BMDCs (TNP-DC) from indicated mice. After 5 days, ear-swelling responses after challenge ( d ) as well as TNP-specific IFN-γ ( e ) and IL-17A ( f ) production by skin dLN T cells were analysed (means±s.d., n =5 per group, **P <0.01 by Student’s t- test). ( g ) CHS in mice carrying DC-specific deletion of CARD9 (DC- CARD9 −/− ), DAP12 (DC- DAP12 −/− ), NLRP3 (DC- NLRP3 −/− ) or MyD88 (DC- MyD88 −/− ) generated by a method indicated in Supplementary Fig. 5 . Chimeric mice were treated twice with DT 1 week apart and were sensitized with TNCB or vehicle on the abdominal skin. On day 5 after sensitization, ear swelling 24 h after challenge was analysed (means±s.d., n =5 per group, **P <0.01 by Student’s t- test). Data are representative of two independent experiments. ( h , i ) Hapten-specific cytokine response of dLN T cells isolated from DC- CARD9 −/− , DC- DAP12 −/− , DC- NLRP3 −/− , DC- MyD88 −/− and their respective control (DC-WT) mice 5 days after epicutaneous sensitization in g . T cells were stimulated in vitro for 3 days with irradiated spleen cells modified with TNP. IFN-γ ( h ) and IL-17A ( i ) production in the culture was measured by ELISA (means±s.d., n =5 per group, **P <0.01 by Student’s t- test). Full size image Skin exposure to contact allergens induces release of inflammatory cytokines including IL-1α/β from keratinocytes, which was also reported to play a role in the sensitization process of CHS [27] , [39] . Thus, the intradermal injection of TNP-DCs might not reflect the milieu that occurs in the skin upon hapten application. To clarify the role for DAP12-CARD9 signal activation and IL-1 production in skin DCs upon percutaneous sensitization with haptens, we generated mice carrying DC-specific deletion of CARD9, DAP12, NLRP3 or MyD88 (DC- CARD9 −/− , DC- DAP12 −/− , DC- NLRP3 −/− or DC- MyD88 −/− mice, respectively) by a method that combines a mixed bone marrow chimera with the diphtheria toxin (DT) receptor (DTR)-mediated conditional cell knockout (Treck) system [40] ( Supplementary Fig. 5 ). For the generation of DC- CARD9 −/− mice, we reconstituted lethally irradiated recipient mice with a 1:1 mixture of bone marrow cells from CARD9 −/− mice and those from Ly5.1 congenic CD11c-DTR Tg mice, which express DTR under the control of CD11c promoter [41] . In the chimeric mice, only the Ly5.1 + Ly5.2 – CD11c + DCs originating from CD11c-DTR Tg mice were positive for DTR. Therefore, DT treatment specifically depleted Ly5.1 + Ly5.2 – DCs but not Ly5.1 – Ly5.2 + CARD9 −/− DCs, resulted in a CARD9-deficient condition only in DCs ( Supplementary Fig. 5 ) in the circulation (spleen) ( Supplementary Fig. 6a ) as well as in the skin ( Supplementary Fig. 6b ). In contrast, CD11c − hematopoietic cells, such as CD3 + CD4 + and CD8 + CD3 + T cells, CD19 + B cells, CD11c − Ly6G + neutrophils and CD11c-CD11b + macrophages, were not affected by DT treatment irrespective of the genotype of donor cells. The control mice (DC-WT) were reconstituted with a mixture of bone marrow cells from Ly5.2 congenic CARD9 −/− CD11c-DTR Tg mice and Ly5.1 congenic WT mice, resulting in the deletion of only Ly5.1 − Ly5.2 + CARD9 −/− DCs but not Ly5.1 + Ly5.2 – WT DCs after DT treatment. Note that we used Lang-DTREGFP mice, which express the DTR in epidermal LCs [42] , as recipients in this system so as to enable depletion of radio-resistant LCs by DT treatment. Thus, skin DCs in DT-treated chimeric mice were depleted of LCs with dermal DCs being replaced by donor cells. It has been shown previously that depletion of LCs in Lang-DTREGFP mice does not affect CHS [42] . We generated DC- DAP12 −/− , DC- NLRP3 −/− or DC- MyD88 −/− mice and their respective control mice by the same way. We epicutaneously sensitized these DT-treated chimeric mice with TNCB and assessed the CHS reaction. We found that DC- CARD9 −/− , DC- DAP12 −/− or DC- NLRP3 −/− mice, but not DC- MyD88 −/− mice, exhibited markedly reduced CHS responses relative to their control mice ( Fig. 3g and Supplementary Fig. 7a–d ) due to defective development of hapten-reactive T cells in the skin dLNs ( Fig. 3h,i ). These data suggest that lack of CARD9, DAP12 or NLRP3 signal in skin DCs is sufficient to abolish CHS induction. Together, DAP12-CARD9 signalling and the NLRP3 inflammasome control IL-1α and IL-1β secretion by DCs after hapten stimulation and these processes are essential for CHS induction by DCs. ITAM-Syk signal controls hapten-induced caspase-1 activation Next, we examined the mechanisms by which haptens engage the NLRP3 inflammasome. We assessed intracellular caspase-1 activity with a fluorescence probe, 5-carboxyfluorescein-YVAD-fmk (FAM-YVAD-fmk). After TNBS or ATP treatment, a large proportion of BMDCs increased fluorescence intensity relative to untreated controls, which indicated the intracellular generation of active caspase-1 ( Fig. 4a ). Common mechanisms implicated in NLRP3 inflammasome activation include potassium (K + ) efflux, lysosomal damage with release and activation of cathepsin B and ROS production [43] . To determine the role of these intermediary signals, we used pharmacological inhibitors to block specific signalling pathways. We found that similar to activation by ATP, TNBS-induced caspase-1 activation was almost completely blocked by the potassium channel blocker glibenclamide or by the ROS inhibitors N -acetyl- L -cysteine (NAC) or (2R,4R)-4-aminopyrrolidine-2,4-dicarboxylate (APDC) ( Fig. 4a ). However, blockade of the lysosomal cathepsin B pathway by the lysosomal acidification inhibitor bafilomycin A did not influence caspase-1 activation. Inhibition of the ATP receptor P2X 7 by KN-62 partially attenuated the caspase-1 activation induced by TNBS, which may support a previous report that P2X 7 -deficient DCs fail to induce CHS [15] . In addition, Syk inhibitor BAY61-3606 almost completely blocked caspase-1 activation by TNBS but not ATP, which indicates that Syk specifically controls the pathway for inflammasome activation by TNBS. Together, these data suggest that hapten-induced activation of caspase-1 is dependent on K + efflux, ROS production and Syk activity, but not on lysosomal damage. 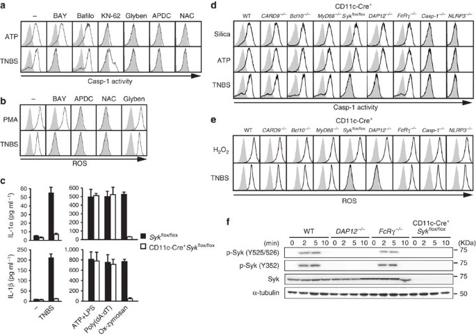Figure 4: DAP12-Syk signalling controls contact allergen-induced ROS production and caspase-1 activation. (a) Caspase-1 (Casp-1) activation in BMDCs left untreated (−) or pretreated with BAY61-3606 (BAY; 3 μM), bafilomycin A (bafilo; 100 nM), KN-62 (10 μM), Glibenclamide (Gliben; 25 μM), APDC (50 μM) or NAC (10 μM) and stimulated with ATP (5 mM) or TNBS (100 μg ml−1) for 8 h. After the stimulation, cells were incubated with FAM-YVAD-FMK and fluorescence intensity was analysed by flow cytometry gating on PI−live cells. Gray-filled histograms: unstimulated control cells. (b) Intracellular ROS production in BMDCs left untreated (−) or pretreated with indicated inhibitors as in A, followed by stimulation with PMA (10 ng ml−1) or TNBS (100 μg ml−1) in the presence of CM-H2DCFDA. Fluorescence was analysed by flow cytometry gating on PI−live cells. Gray-filled histograms: unstimulated control cells. (c) IL-1α and IL-1β secretion by BMDCs fromSykfox/floxand CD11c-Cre+Sykflox/floxmice after stimulation with TNBS (100 μg ml−1) (means±s.d.,n=3 per group). (d) Casp-1 activation. BMDCs from indicated mice were stimulated with silica (100 μg ml−1), ATP (5 mM) or TNBS (100 μg ml−1) for 8 h and incubated with FAM-YVAD-FMK. Fluorescence intensity was analysed by flow cytometry gating on PI−live cells. Gray-filled histograms: unstimulated control cells. (e) Intracellular ROS production. BMDCs from indicated mice were stimulated with H2O2(100 μM) or TNBS (100 μg ml−1) in the presence of CM-H2DCFDA. The fluorescence intensity was analysed by flow cytometry gating on CD11c+PI−cells. Gray-filled histograms: unstimulated control cells. (f) Syk activation in WT,DAP12−/−,FcRγ−/−and CD11c-Cre+Sykflox/floxBMDCs stimulated with TNBS (100 μg ml−1) for the indicated times. Cell lysates were analysed by immunoblotting for phosphorylated-Syk (Tyr525/526 or Tyr352), total Syk and α-tubulin. α-Tubulin is an internal control for total protein loading. Figure 4: DAP12-Syk signalling controls contact allergen-induced ROS production and caspase-1 activation. ( a ) Caspase-1 (Casp-1) activation in BMDCs left untreated (−) or pretreated with BAY61-3606 (BAY; 3 μM), bafilomycin A (bafilo; 100 nM), KN-62 (10 μM), Glibenclamide (Gliben; 25 μM), APDC (50 μM) or NAC (10 μM) and stimulated with ATP (5 mM) or TNBS (100 μg ml −1 ) for 8 h. After the stimulation, cells were incubated with FAM-YVAD-FMK and fluorescence intensity was analysed by flow cytometry gating on PI − live cells. Gray-filled histograms: unstimulated control cells. ( b ) Intracellular ROS production in BMDCs left untreated (−) or pretreated with indicated inhibitors as in A, followed by stimulation with PMA (10 ng ml −1 ) or TNBS (100 μg ml −1 ) in the presence of CM-H2DCFDA. Fluorescence was analysed by flow cytometry gating on PI − live cells. Gray-filled histograms: unstimulated control cells. ( c ) IL-1α and IL-1β secretion by BMDCs from Syk fox/flox and CD11c-Cre + Syk flox/flo x mice after stimulation with TNBS (100 μg ml −1 ) (means±s.d., n =3 per group). ( d ) Casp-1 activation. BMDCs from indicated mice were stimulated with silica (100 μg ml −1 ), ATP (5 mM) or TNBS (100 μg ml −1 ) for 8 h and incubated with FAM-YVAD-FMK. Fluorescence intensity was analysed by flow cytometry gating on PI − live cells. Gray-filled histograms: unstimulated control cells. ( e ) Intracellular ROS production. BMDCs from indicated mice were stimulated with H 2 O 2 (100 μM) or TNBS (100 μg ml −1 ) in the presence of CM-H 2 DCFDA. The fluorescence intensity was analysed by flow cytometry gating on CD11c + PI − cells. Gray-filled histograms: unstimulated control cells. ( f ) Syk activation in WT, DAP12 −/− , FcRγ −/− and CD11c-Cre + Syk flox/flox BMDCs stimulated with TNBS (100 μg ml −1 ) for the indicated times. Cell lysates were analysed by immunoblotting for phosphorylated-Syk (Tyr525/526 or Tyr352), total Syk and α-tubulin. α-Tubulin is an internal control for total protein loading. Full size image Next, we examined factors that regulate ROS production by TNBS. Intracellular ROS levels were determined using the ROS-sensitive probe CM-H 2 DCFDA, which produces a fluorogenic product upon oxidation. ROS production was significantly increased after TNBS or PMA treatment relative to untreated controls and was blocked by APDC or NAC ( Fig. 4b ). Treatment of BMDCs with the Syk inhibitor almost completely inhibited the ROS production induced by TNBS but not PMA, which indicates that Syk specifically controls hapten-induced ROS production ( Fig. 4b ). In contrast to caspase-1 activation, treatment with glibenclamide did not influence TNBS-induced ROS production, which indicates that K + efflux functions downstream or independently of Syk-dependent ROS production for inflammasome activation. Consistent with the dependency of caspase-1 activation and ROS production on Syk, IL-1α/β secretion after stimulation with TNBS was almost completely abrogated in BMDCs from DC-conditional Syk-deficient mice (CD11c-Cre + Syk flox/flox ) ( Fig. 4c ). Thus, Syk controls hapten-induced ROS production required for NLRP3 inflammasome activation. Next, we examined whether DAP12, FcRγ, MyD88, CARD9 and BCL10 were involved in Syk-regulated ROS production and inflammasome activation after hapten stimulation. As expected, loss of NLRP3 abolished caspase-1 activation by TNBS as well as ATP and silica, but did not influence ROS production caused by these stimuli. As Syk deficiency, loss of DAP12, but not FcRγ, abrogated both caspase-1 activation ( Fig. 4d ) and ROS production ( Fig. 4e ) induced by TNBS, but not by ATP or silica. We found that TNBS stimulation in vitro significantly increased Syk phosphorylation in WT BMDCs similarly to the increase induced by ox-zymosan ( Supplementary Fig. 8 ). However, the TNBS-induced Syk activation was completely abolished in DAP12 −/− but not FcR γ −/− BMDCs ( Fig. 4f and Supplementary Fig. 10a ). These data indicate that DAP12 controls Syk activation and therefore is essential for ROS production and inflammasome activation induced by hapten stimulation. CARD9/BCL10 controls pro-IL-1α/β induction regulated by NF-κB In contrast to Syk or DAP12 deficiency, neither TNBS-induced ROS production nor caspase-1 activation was affected by the loss of CARD9 or BCL10 ( Fig. 4d,e ), despite these deficiency-abrogated IL-1α/β secretions, which indicates that the CARD9/BCL10 complex is not involved in inflammasome activation. Given that the CARD9/BCL10 complex regulates ITAM-coupled receptor-mediated NF-κB activation [28] , we examined whether CARD9-mediated signalling was required for synthesis of pro-IL-1α/β regulated by NF-κB activation. We found that intracellular pro-IL-1α and -1β levels after stimulation with TNBS but not LPS+ATP were markedly reduced in CARD9 −/− , BCL10 −/− , Syk −/− and DAP12 −/− BMDCs relative to WT BMDCs ( Fig. 5a ). In contrast, deletion of MyD88, FcRγ, NLRP3 and caspase-1 had no effect on the IL-1α/β synthesis. Nuclear translocation of NF-κBp65 and NF-κBc-Rel after TNBS stimulation was almost completely abolished in CARD9 −/− BMDCs ( Fig. 5b and Supplementary Fig. 10b ). Moreover, priming of cells with LPS, which activates NF-κB through TLR4 independent of Syk, restored the defective TNBS-induced production of IL-1β by CARD9 −/− and BCL10 −/− BMDCs ( Fig. 5c ). Therefore, signalling through CARD9/BCL10 selectively controls signal 1 for IL-1α/β secretion by regulating hapten-induced NF-κB activation, while DAP12-Syk signalling is required for both signal 1 and signal 2. 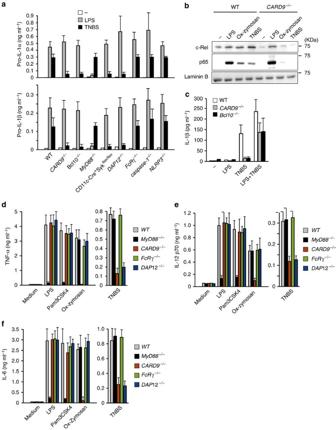Figure 5: CARD9/BCL10 selectively controls NF-κB activation required for pro-IL-1α/β synthesis. (a) Pro-IL-1α and pro-IL-1β levels in BMDCs from indicated mice stimulated with TNBS (100 μg ml−1) or LPS (1 ng ml−1) for 12 h in the presence of z-VAD-fmk (100 μM). Cells were lysed in hypotonic buffer and intracellular pro-IL-1α and pro-IL-1β levels were determined by ELISA (means±s.d.,n=3 per group). (b) Immunoblotting of NF-κB, c-Rel, p65 and lamin B in the nuclear extracts of WT andCARD9−/−BMDCs stimulated with LPS (10 ng ml−1), ox-zymosan (100 μg ml−1) or TNBS (100 μg ml−1). The nuclear protein lamin B served as a loading control. Representative data of three independent experiments were shown. (c) IL-1β secretion by WT,CARD9−/−andBCL10−/−BMDCs stimulated with LPS (1 ng ml−1) or TNBS (100 μg ml−1) or with TNBS after LPS priming. DAP12-CARD9 signalling pathway is crucial for cytokine response of DCs to TNBS (means±s.d.,n=3 per group). (d–f) Production of TNF-α (d), IL-12p70 (e) and IL-6 (f) by WT,MyD88−/−,CARD9−/−,FcRγ−/−orDAP12−/−BMDCs after stimulation with LPS (10 ng ml−1), Pam3CSK4 (100 ng ml−1), Ox-zymosan (100 μg ml−1) or TNBS (100 μg ml−1) for 24 h (means±s.d.,n=3 per group). Figure 5: CARD9/BCL10 selectively controls NF-κB activation required for pro-IL-1α/β synthesis. ( a ) Pro-IL-1α and pro-IL-1β levels in BMDCs from indicated mice stimulated with TNBS (100 μg ml −1 ) or LPS (1 ng ml −1 ) for 12 h in the presence of z-VAD-fmk (100 μM). Cells were lysed in hypotonic buffer and intracellular pro-IL-1α and pro-IL-1β levels were determined by ELISA (means±s.d., n =3 per group). ( b ) Immunoblotting of NF-κB, c-Rel, p65 and lamin B in the nuclear extracts of WT and CARD9 −/− BMDCs stimulated with LPS (10 ng ml −1 ), ox-zymosan (100 μg ml −1 ) or TNBS (100 μg ml −1 ). The nuclear protein lamin B served as a loading control. Representative data of three independent experiments were shown. ( c ) IL-1β secretion by WT, CARD9 −/− and BCL10 −/− BMDCs stimulated with LPS (1 ng ml −1 ) or TNBS (100 μg ml −1 ) or with TNBS after LPS priming. DAP12-CARD9 signalling pathway is crucial for cytokine response of DCs to TNBS (means±s.d., n =3 per group). ( d – f ) Production of TNF-α ( d ), IL-12p70 ( e ) and IL-6 ( f ) by WT, MyD88 −/− , CARD9 −/− , FcRγ −/− or DAP12 −/− BMDCs after stimulation with LPS (10 ng ml −1 ), Pam3CSK4 (100 ng ml −1 ), Ox-zymosan (100 μg ml −1 ) or TNBS (100 μg ml −1 ) for 24 h (means±s.d., n =3 per group). Full size image Because NF-κB regulates expression of many genes involved in inflammation and cellular activation, we examined whether DAP12-CARD9 signalling controlled the synthesis of pro-inflammatory cytokines, other than IL-1α/β, and DC maturation. Similar to IL-1 production, TNF-α, IL-12p70 and IL-6 productions were markedly impaired in CARD9 −/− and DAP12 −/− BMDCs, but not in FcR γ −/− and MyD88 −/− BMDCs, after TNBS stimulation ( Fig. 5d–f ). Because IL-18 secretion is regulated by inflammasome and was suggested be involved in CHS [25] , we also attempted to measure IL-18 production. However, we could not detect IL-18 in the culture supernatant after TNBS stimulation. Upregulation of the DC maturation markers CD40, CD86, MHC class-II and CCR7 was not significantly influenced by CARD9 deficiency ( Supplementary Fig. 9 ). Thus, the DAP12–CARD9 pathway is crucial for innate cytokine productions by DCs but dispensable for DC maturation after hapten stimulation. Haptens but not irritants can activate Syk-CARD9 signalling Given that our data indicated that the IL-1 was a crucial factor for T-cell priming by DCs and its secretion was regulated by the Syk-CARD9 signalling, we hypothesized that the allergenic properties of chemical compounds might be associated with their capacity to stimulate Syk signalling in DCs. Thus, we examined this capacity in various haptens [fluorescein isothiocyanate (FITC), oxazolone and 2,4-dinitrofluorobenzene (DNFB)] and non-allergenic irritants [SLS, benzoic acid (BA) and methyl salicylate (MS)]. We stimulated BMDCs in vitro with these chemicals and found that all haptens examined were capable of inducing the secretion of both IL-1α and IL-1β by DCs, whereas all irritants examined were incapable of it ( Fig. 6a ). In line with the IL-1α/β production, stimulation with haptens but not irritants induced ROS production ( Fig. 6b ) and caspase-1 activation ( Fig. 6c ) in DCs. In addition, all haptens but not irritants were capable of inducing Syk phosphorylation in DCs ( Fig. 6d and Supplementary Fig. 10c ). Thus, haptens commonly can induce ROS-mediated inflammasome activation and IL-1α/β secretion by activating Syk signalling in DCs. Moreover, similarly in response to TNBS, loss of CARD9 or Syk abolished the production of both IL-1α and IL-1β induced by all these haptens tested ( Fig. 6e ), which suggests that Syk-CARD9 signalling plays a broad and essential role in IL-1α/β responses to haptens. However, although DAP12 is required for IL-1α/β production in response to oxazolone and DNFB, it was dispensable for the response to FITC, which suggests compound specificity in DAP12-dependent responses. Consistent with the requirement for signalling molecules in IL-1α/β secretion, ROS production and caspase-1 activation induced by DNFB and oxazolone were dependent on DAP12 and Syk, whereas ROS production and caspase-1 activation induced by FITC were dependent on Syk but not DAP12 ( Fig. 6f,g ). In contrast, as observed for TNBS, CARD9 was dispensable for both ROS production and caspase-1 activation in response to all of these haptens. 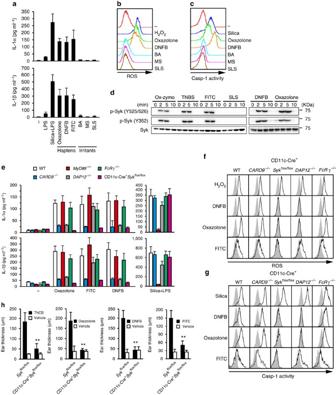Figure 6: Contact allergenicity of chemicals depends on the capacity to trigger Syk signalling. (a) IL-1α and IL-1β secretion by BMDCs after stimulation with LPS (1 ng ml−1), LPS plus silica (100 μg ml−1), oxazolone (10 μg ml−1), dinitrofluorobenzene (DNFB; 100 μg ml−1), FITC (5 μg ml−1), BA (10 μg ml−1), MS (10 μg ml−1) or SLS (5 μg ml−1) (means±s.d.,n=4 per group). (b) Intracellular ROS production. BMDCs were stimulated with H2O2(100 μM) or the indicated contact sensitizers and irritants as inain the presence of CM-H2DCFDA. Fluorescence intensity was analysed by flow cytometry gating on PI−live cells. (c) Casp-1 activation. BMDCs were stimulated with silica or the indicated contact sensitizers and irritants as ina, incubated with FAM-YVAD-FMK, and analysed by flow cytometry gating on PI−live cells. (d) Syk activation in WT BMDCs stimulated with the indicated contact sensitizers and irritants for the indicated times. Cell lysates were analysed by immunoblotting for levels of phosphorylated-Syk (Tyr525/526 or Tyr352) or total Syk. (e) IL-1α and IL-1β secretion by WT,CARD9−/−,MyD88−/−,DAP12−/−,FcRγ−/−orSyk−/−BMDCs stimulated with oxazolone, DNFB or FITC, or with silica after 3-h LPS priming (means±s.d.,n=3 per group). (f) ROS production. BMDCs from indicated mice were stimulated with H2O2, DNFB or oxazolone in the presence of CM-H2DCFDA, or stimulated with FITC in the presence of CellROX Deep Red Reagent, and analysed as inb. Gray-filled histograms: unstimulated cells. (g) Casp-1 activation. BMDCs from indicated mice were stimulated with silica, DNFB, oxazolone or FITC, treated with FAM-YVAD-FMK or 667-YVAD-FMK (for FITC), and analysed as inc. Gray-filled histograms: unstimulated cells. (h) CHS response in DC-specific Syk-deficient mice.Sykflox/floxand CD11c-Cre+Sykflox/floxmice were epicutaneously treated with TNCB, oxazolone, DNFB, FITC or their respective vehicles. On day 5 after sensitization, the ear swelling response 24 h after challenge was analyzed (means±s.d.,n=5 per group,**P<0.01 by Student’st-test). Data are representative of two or three independent experiments. Figure 6: Contact allergenicity of chemicals depends on the capacity to trigger Syk signalling. ( a ) IL-1α and IL-1β secretion by BMDCs after stimulation with LPS (1 ng ml −1 ), LPS plus silica (100 μg ml −1 ), oxazolone (10 μg ml −1 ), dinitrofluorobenzene (DNFB; 100 μg ml −1 ), FITC (5 μg ml −1 ), BA (10 μg ml −1 ), MS (10 μg ml −1 ) or SLS (5 μg ml −1 ) (means±s.d., n =4 per group). ( b ) Intracellular ROS production. BMDCs were stimulated with H 2 O 2 (100 μM) or the indicated contact sensitizers and irritants as in a in the presence of CM-H 2 DCFDA. Fluorescence intensity was analysed by flow cytometry gating on PI − live cells. ( c ) Casp-1 activation. BMDCs were stimulated with silica or the indicated contact sensitizers and irritants as in a , incubated with FAM-YVAD-FMK, and analysed by flow cytometry gating on PI − live cells. ( d ) Syk activation in WT BMDCs stimulated with the indicated contact sensitizers and irritants for the indicated times. Cell lysates were analysed by immunoblotting for levels of phosphorylated-Syk (Tyr525/526 or Tyr352) or total Syk. ( e ) IL-1α and IL-1β secretion by WT, CARD9 −/− , MyD88 −/− , DAP12 −/− , FcRγ −/− or Syk −/− BMDCs stimulated with oxazolone, DNFB or FITC, or with silica after 3-h LPS priming (means±s.d., n =3 per group). ( f ) ROS production. BMDCs from indicated mice were stimulated with H 2 O 2 , DNFB or oxazolone in the presence of CM-H2DCFDA, or stimulated with FITC in the presence of CellROX Deep Red Reagent, and analysed as in b . Gray-filled histograms: unstimulated cells. ( g ) Casp-1 activation. BMDCs from indicated mice were stimulated with silica, DNFB, oxazolone or FITC, treated with FAM-YVAD-FMK or 667-YVAD-FMK (for FITC), and analysed as in c . Gray-filled histograms: unstimulated cells. ( h ) CHS response in DC-specific Syk-deficient mice. Syk flox/flo x and CD11c-Cre + Syk flox/flox mice were epicutaneously treated with TNCB, oxazolone, DNFB, FITC or their respective vehicles. On day 5 after sensitization, the ear swelling response 24 h after challenge was analyzed (means±s.d., n =5 per group, **P <0.01 by Student’s t- test). Data are representative of two or three independent experiments. Full size image Finally, to investigate the importance of Syk signalling in skin DCs upon percutaneous immunization with haptens in vivo , we epicutaneously sensitized DC-conditional Syk-deficient (CD11c-Cre + Syk flox/flox ) mice with various haptens and examined the CHS response. CD11c-Cre + Syk flox/flox mice displayed a markedly reduced CHS response to all examined haptens relative to control Syk flox/flox mice ( Fig. 6h ). These indicate a broadly essential role for Syk signalling in skin DCs in the sensitization of CHS. Therefore, these data suggest that the ability to activate Syk signalling, which provides sufficient signals for IL-1α/β secretion by DCs, seems to be a general property of haptens associated with their allergenicity. In the current study, we have identified that IL-1 production by DCs induced by haptens requires ITAM-Syk-mediated NLRP3 inflammasome activation and Syk-CARD9/BCL10-mediated pro-IL-1 synthesis. ATP is released from damaged or dying cells and engages NLRP3 inflammasome through activation of the purinergic receptor P2X 7 (ref. 44 ). It has been shown that a P2X 7 deficiency abrogates the sensitization capacity of BMDCs [15] . We found that the inhibition of P2X 7 by a specific blocker dampens the caspase-1 activation induced by hapten, which suggests that ATP and P2X 7 contribute to the Syk-mediated inflammasome activation pathway. Because we also found that hapten-induced NLRP3 inflammasome activation is dependent on ROS production and K + efflux, it is likely that P2X 7 acts as an ion channel to efflux K + in response to Syk-mediated ROS production. A previous report suggested that IL-1α, rather than IL-1β, plays a crucial role in CHS development [22] . In contrast to IL-1β secretion, which is strictly dependent on inflammasomes, IL-1α secretion is not always dependent on the inflammasome. For example, whereas IL-1α secretion in response to ATP, nigericin or Candida albicans was dependent on the NLRP3 inflammasome, IL-1α was released independently of the NLRP3 inflammasome in response to particulate activators such as MDU, alum or silica [45] . We found that TNBS stimulation also induced substantial secretion of IL-1α by DCs, and this secretion was completely dependent on NLRP3, which suggests that hapten-induced IL-1α secretion is regulated by a mechanism similar that utilized for ATP, nigericin and C. albicans . We identified that the ITAM-Syk-CARD9 pathway is an essential innate signalling in DCs to initiate contact sensitization to haptens. Martin et al . [11] reported that DCs lacking both TLR2 and TLR4, but not TLR2 or TLR4 alone, failed to induce CHS. In the absence of IL-12R signalling, however, the absence of TLR4 alone is sufficient to prevent CHS. These data suggest that both an IL-12-independent mechanism, which requires both TLR2/4 activation, and an IL-12-dependent one, which requires only TLR4 activation, are involved in contact sensitization. TLR4 may be activated in vivo by endogenous ligands such as low-molecular weight derivatives of hyaluronic acid [13] , [14] . We found that haptens directly induce cytokine production, including IL-1 and IL-12, dependent on ITAM-CARD9 but not MyD88 in vitro in the absence of hyaluronic acid. These results suggest that the ITAM-signalling controls the IL-12-dependent mechanism, while TLR2/4-MyD88 signalling controls the IL-12-independent one triggered by the hapten stimulation in skins. A recent report has shown that type I interferon signalling mediated through the TLR4-TRIF pathway is involved in NLRP3 inflammasome activation in response to gram-negative bacteria [46] . This may suggest the possibility of cross-talk and/or synergy between the ITAM-Syk-mediated and the TLR4-TRIF-mediated pathways for NLRP3 inflammasome activation. Our data clearly showed that Syk-coupled signalling plays an essential role in detecting various haptens and activating the innate immune system to sensitize CHS. In addition, the responses to chemical allergens other than FITC required DAP12. Although we did not identify specific receptors in this study, our data implicate the presence of ITAM-coupled receptors sensing haptens. Whereas DAP12 signal dependency or independency for various sensitizers may indicate the presence of receptors that recognize different structure of haptens, Syk-coupled receptors may sense common signals derived from tissue/cell damage caused by haptens. For instance, the ITAM-coupled CLRs CLEC9A and Mincle recognize F-actin and spliceosome-associated protein 130 (SAP130) released from necrotic cells, respectively [47] , [48] , [49] . Alternatively, Syk may sense haptens in a receptor-independent manner as suggested for the recognition of MSU crystals, which may involve aggregation of cell membrane cholesterol through mechanisms that are incompletely understood [50] . It should also be explored whether the ability to activate Syk signalling is associated with the ability to haptenize proteins. Previous studies have shown that other types of skin allergens and fungi associated with skin inflammation are also recognized by ITAM-coupled receptors. For example, the FcRγ-associated CLR Dectin-2 recognizes the house dust mite Dermatophagoides farinae [51] , whose products are highly allergic and associated with severe eczema in atopic dermatitis. This recognition mediates Th2 immunity to Dermatophagoides farinae through the generation of cysteinyl leukotrienes. Activation of CARD9 signalling through recognition by Dectin-1 and Dectin-2 are essential for the host defence against C. albicans [32] , [33] , [34] . Recognition of C. albicans induces IL-1β secretion by DCs with signalling mechanisms similar to those used in response to chemical sensitizers: caspase-1 activation through the Dectin-1-Syk-ROS-NLRP3 signalling pathway and pro-IL-1β synthesis dependent on NF-κB activation through the Syk-CARD9/BCL10 signalling pathway [33] . IL-1β released by this pathway is involved in the differentiation of protective Th17 cells for anti- Candida defence. A FcRγ-associated CLR, Mincle, recognizes the Malassezia species, which are associated with several skin diseases such as tinea versicolor, folliculitis and atopic dermatitis [52] . A recent study reported that stimulation of Mincle by the ligand trehalose-6,6′-dibehenate induces CARD9- and NLRP3 inflammasome-dependent IL-1β secretion from BMDCs [53] . Thus, the ITAM-Syk-CARD9-IL-1 pathway appears to play a general role in the pathogenesis of inflammatory skin diseases, and the capacity to trigger this pathway may determine the pathogenicity of allergens and microorganisms. In conclusion, we identified that ITAM-Syk-CARD9 signalling is essential for IL-1α/β secretion by DCs in response to various haptens. In addition to the ‘first signal’ delivered through TCRs by the MHC:self peptide–hapten complex, IL-1s secreted by hapten-activated DCs delivers an essential ‘second signal’ to naïve T cells for their differentiation into effector T cells in dLNs ( Fig. 7 ). Therefore, this study provides new perspectives for prophylaxis and control of ACD. 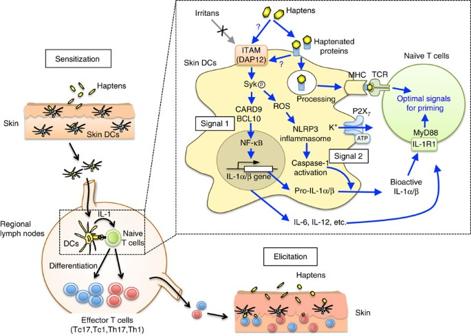Figure 7: DC activation through ITAM-Syk-CARD9 signalling is required for the priming of hapten-specific T cells. Haptens, but not irritants, can ‘haptenize’ proteins to form a hapten self-protein complex, which is eventually presented by DCs as an altered-self antigen to trigger TCRs. In addition, haptens but not irritants have the capacity to activate ITAM-Syk signalling in DCs. Syk activation not only induces the CARD9/BCL10-regulated NF-κB activation required for the intracellular synthesis of pro-IL-1α/β (SIGNAL 1), but also induces ROS generation required for NLRP3 inflammasome activation (SIGNAL 2). K+efflux and P2X7 also contribute to inflammasome activation. As a result, bioactive IL-1α/β are secreted by antigen-presenting DCs, which in turn stimulates naïve T cells through the IL-1R1-Myd88 pathway, delivering essential additional signals required for the priming of hapten-specific T cells in the dLNs. CARD9/BCL10-regulated NF-κB activation is also required for hapten-induced IL-6 and IL-12 production that drives effector T-cell differentiation. Figure 7: DC activation through ITAM-Syk-CARD9 signalling is required for the priming of hapten-specific T cells. Haptens, but not irritants, can ‘haptenize’ proteins to form a hapten self-protein complex, which is eventually presented by DCs as an altered-self antigen to trigger TCRs. In addition, haptens but not irritants have the capacity to activate ITAM-Syk signalling in DCs. Syk activation not only induces the CARD9/BCL10-regulated NF-κB activation required for the intracellular synthesis of pro-IL-1α/β (SIGNAL 1), but also induces ROS generation required for NLRP3 inflammasome activation (SIGNAL 2). K + efflux and P 2 X7 also contribute to inflammasome activation. As a result, bioactive IL-1α/β are secreted by antigen-presenting DCs, which in turn stimulates naïve T cells through the IL-1R1-Myd88 pathway, delivering essential additional signals required for the priming of hapten-specific T cells in the dLNs. CARD9/BCL10-regulated NF-κB activation is also required for hapten-induced IL-6 and IL-12 production that drives effector T-cell differentiation. Full size image Mice All mice used in this study were female and between the ages of 7–12 weeks. C57BL/6 and BALB/c mice were purchased from Kyudo. CARD9 −/− mice were generated previously as described [28] and backcrossed onto C57BL/6 or BALB/c mice over eight times. BCL10 −/− , Caspase-1 −/− , MyD88 −/− , DAP12 −/− , Rag2 −/− , FcR γ −/− , Syk flox/flox , Langerin-DTREGFP knock-in ( Lang-DTREGFP ), CD11c-DTR transgenic (Tg) were generated previously as described [41] , [42] , [54] , [55] , [56] , [57] , [58] , [59] , [60] . CD11c-Cre Tg mice were purchased from Jackson Laboratory (Bar Harbor, ME). C57BL/6-Ly5.1 congenic mice were purchased from Sankyo Labo Service (Tokyo, Japan). IL-1R1 −/− mice were provided by Immunex [61] . NLRP3 −/− mice were provided by Genentech (South San Francisco, CA). CD11c-Cre + Syk flox/flo x mice were generated by crossing Syk flox/flox mice with CD11c-Cre Tgmice. All experiments were approved by the Institutional Animal Research Committee of Saga University and animals were treated in accordance with the ethical guidelines of Saga University. Antibodies and reagents Antibodies specific for Syk (2712), p-Syk (Tyr525/526) (2711) and p-Syk (Tyr352) (2701) were from Cell Signaling; α-tubulin (DM1A) antibody was from Sigma; NF-κB p65 (sc-372), c-Rel (sc-71) and lamin B (sc-6217) antibodies were from Santa Cruz Biotechnology; Thy1.2 (53.2.1), CD16/CD32 (2.4G2), Ly5.1/CD45.1 (A20), Ly5.2/CD45.2 (104), CD3ε (145-2C11), CD19 (1D3), CD4 (L3T4), CD8a (53.6.7), CD11b/Mac1 (M1/70), CD11c (N418), Ly6G (RB6-8C5), CD62L (MEL-14), CCR7 (4B12), I-A b (AF6-120.1), CD80 (16-10A1), CD86 (GL1), CD40 (3/23) and IL-17A (eBio17B7) antibodies were from eBioscience and BD Biosciences. Phorbol 12-myristate 13-acetate (PMA), calcium ionophore A231877, TNCB, 2,4,6-trinitrobenzenesulfonic acid (TNBS), DNFB, FITC, oxazolone BA, MS, (SLS), DT (D0564), ovalbumin, propidium iodide (PI), bafilomycin A, KN-62, glibenclamide, N -acetyl-cysteine (NAC), (2R,4R)-4-aminopyrrolidine-2,4-dicarboxylic acid (APDC), hyaluronidase, DNase I, DMEM medium and RPMI 1640 medium were from Sigma. Liberase TM was from Roche. BAY61-3606 was from Calbiochem. Fetal bovine serum (FBS) was from Hyclone. 2-Mercaptoethanol was from Gibco. ATP (017-21511) was from Wako Biochemicals. [ 3 H]-thymidine was from Amersham. Penicillin/streptomycin was from Nacalai Tesque. Recombinant GM-CSF was from Peprotech. Ultrapure LPS, Poly (dA:dT), and Pam3CSK4 were from Invivogen. NaClO-oxidized zymosan (ox-zymosan) was prepared as reported previously [62] . In brief, Zymosan (1 g) was suspended for 1 d at 4 °C in 100 ml of 0.1 M NaOH with 0.5% NaClO. The insoluble fraction (NaClO-oxidized zymosan) was then collected by centrifugation and was suspended in 1 ml of saline and was sonicated for 30 s. Silica (average grain diameter 1–2 μm) was prepared as reported previously [63] . CM-H 2 DCFDA was from Molecular Probes. CellROX Deep Red Dye was from Invitrogen. FAM-YVAD-fmk and 660-YVAD-fmk were from Immunochemistry Technologies. Z-VAD-fmk was from R&D Systems. ELISA kits for murine IL-1α, IL-1β, IFN-γ, IL-17A, TNF, IL-6 and IL-12p70 were from R&D Systems and eBioscience and were used according to the manufacturer’s instructions. ELISA data are depicted as the mean±s.d. of triplicates. Contact hypersensitivity For induction of CHS to TNCB, mice were sensitized by painting 100 μl of 7% TNCB in acetone, or acetone alone as vehicle control, on the shaved abdomen as previously described [3] . Alternatively, mice were sensitized by intracutaneous injection of 3 × 10 5 TNP-modified bone marrow-derived DCs (TNP-DCs) in 50 μl of phosphate-buffered saline (PBS) into two sites of the shaved abdomen as previously described [35] . Five days after sensitization, mice were challenged on each side of both ears by applying 20 μl of 1% TNCB. For induction of CHS to DNFB, mice were sensitized by painting 100 μl of 0.5% DNFB in ethanol, or ethanol alone as vehicle control, on the shaved abdomen as previously described [64] . Five days after sensitization, mice were challenged on each side of both ears by applying 20 μl of 0.2% DNFB. For induction of CHS to oxazolone, mice were sensitized by painting 100 μl of 2% oxazolone in ethanol, or ethanol alone as vehicle control, on the shaved abdomen as previously described [64] . Five days after sensitization, mice were challenged on each side of both ears by applying 20 μl of 1% oxazolone. For induction of CHS to FITC, mice were sensitized by painting 100 μl of 0.2% FITC in 1:1 acetone/dibutyl phthalate (Ac/DBP), or 1:1 Ac/DBP alone as vehicle control, on the shaved abdominal skin as described previously [11] . Six days after sensitization, mice were challenged on each side of both ears by applying 20 μl of 0.2% FITC/Ac/DB. Ear swelling was measured using an engineer's micrometer (Mitutoyo) 24 h after challenge. Adoptive transfer of CHS Adoptive CHS was performed as previously reported [11] . In brief, mice of the various donor strains were sensitized by painting on the shaved abdominal skin with 100 μl of 7% TNCB/acetone and on both ears with 20 μl of 1% TNCB/acetone. Five days after sensitization, the dLNs (axillary, inguinal and cervical) were harvested and single-cell suspensions were prepared. Thy1.2 + whole T cells were purified from the lymph node cells by positive sorting with a magnetic-activated cell sorting system (MACS; Miltenyi Biotech); the purity was over 95% Thy1.2 + cells as determined by flow cytometry. The purified T cells (1 × 10 7 per mouse) were injected intravenously into naive WT B6-recipient mice. Twenty-four hours after adoptive T-cell transfer, mice were challenged on each side of both ears by applying 20 μl of 1.0% TNCB/acetone, and ear swelling 24 h after the challenge was measured. Ear swelling was determined as the mean difference in ear thickness before and after challenge. Irritant dermatitis Irritant dermatitis was generated as previously reported [65] . In brief, mice received 25 μl of 10% SLS dissolved in dimethylformamide (DMF) on the dorsal and ventral surfaces of the right ear and DMF alone on the left ear. Twenty-four hours later, ear swelling was determined as the mean difference in ear thickness before and after irritant application. Histology Ears from vehicle- or allergen-sensitized mice were removed 24 h after allergen ear challenge and fixed in 4% PBS-buffered paraformaldehyde (Wako Biochemicals); 4-μm organ slices were then prepared and stained with hematoxylin and eosin. DC-specific gene deletion For generating DC-specific deletion of CARD9, MyD88, DAP12 or NLRP3 genes, bone marrow cell suspensions prepared from CARD9 −/− , MyD88 −/− , DAP12 −/− or NLRP3 −/− mice expressing Ly5.2 and WT CD11c-DTR Tg mice congenic for Ly5.1 were mixed 1:1 and intravenously injected (5 × 10 6 cells per mouse) into Lang-DTREGFP mice that had received lethal irradiation (1,000 rad). For controls, bone marrow cell suspensions prepared from CD11c-DTR Tg mice with a CARD9 −/− , MyD88 −/− , DAP12 −/− or NLRP3 −/− background expressing Ly5.2 and WT mice congenic for Ly5.1 were mixed 1:1 and used for transplantation. At least six weeks after transplantation, 2 μg of DT was intraperitoneally administered twice into the chimeric mice 1 week apart. Depletion of DTR + CD11c + DCs in the spleen and ear skin suspensions was analysed using a flow cytometer. Twenty-four hours after the last DT treatment, mice were subjected to CHS experiments. Preparation of cells and fluorescence-activated cell sorting analysis Skin cell suspensions were prepared as described previously [66] . In brief, samples of ear tissue were cut into small pieces and digested in 1 ml of DMEM containing 20 mM HEPES, 0.025 mg ml −1 Liberase TM, 396 U ml −1 DNase I and 0.5 mg ml −1 hyaluronidase at 37 °C for 2 h. Samples were passed through a 40-μm cell strainer, and the cell suspension was washed twice with PBS. For flow cytometry, single-cell suspensions of the skin and spleen were resuspended in PBS/2% bovine serum albumin, FcR blocked with anti-CD16/CD32 (1:100) for 15 min on ice and stained with FITC-, PE-, APC- or PerCP Cy5.5-conjugated Abs (1:100). The Abs used were against Ly5.1, Ly5.2, CD3ε, CD4, CD8α, CD19, CD11c, CD11b and Ly6G. The stained cells were analysed using a FACSCalibur flow cytometer (BD Biosciences) and FlowJo software (TreeStar). In vitro T-cell differentiation Thy1.2 + CD62L high naïve whole T cells isolated from the lymph nodes of WT C57BL/6J, MyD88 −/− or IL-1R1 −/− mice by using a fluorescence-activated cell sorting (FACS) cell sorter (AriaII, BD Biosciences) were co-cultured with WT C57BL/6J, MyD88 −/− or CARD9 −/− BMDCs that were modified with TNP or stimulated with LPS+ATP or ox-zymosan in the presence or absence of 1 μg ml −1 of anti-mouse CD3ε antibody. After 4 days of culture, T cells were collected and re-stimulated for 6 h with PMA (50 ng ml −1 ) plus the calcium ionophore A23187 (1 μM). The supernatants were measured for the concentration of IL-17A and IFN-γ using ELISA. Intracellular expression of IL-17 in the T cells was analysed using a Cytofix/Cytoperm Kit Plus (with Golgistop; BD Biosciences) according to the manufacturer’s instructions. In brief, cells were stimulated with PMA, calcium ionophore and Golgistop for 4 h at 37 °C and labelled with APC-conjugated mouse CD4 or CD8 antibody (1:100). After cells were permeabilized with Cytofix/Cytoperm solution, intracellular cytokine staining was performed using PE-conjugated anti-mouse IL-17A (1:100) and analysed using FACS. Preparation and in vitro stimulation of BMDCs BMDCs were prepared as described previously [67] . In brief, BM cells prepared from femurs and tibias were cultured for 9 days in RPMI 1640 medium supplemented with 10% FBS, 50 μM 2-mercaptoethanol, 50 U ml −1 penicillin, 50 μg ml −1 streptomycin and 20 ng ml −1 GM-CSF. The purity of CD11c-positive cells was higher than 90%. Deletion of the Syk gene in BMDCs from CD11c-Cre + Syk flox/flox was confirmed by western blot analysis of the cell lysate using an anti-mouse Syk antibody. For TNP modification of BMDCs, cells were incubated with 1 mg ml −1 TNBS in RPMI 1640 medium for 7 min at 37 °C, washed three times and resuspended in PBS for CHS immunization. For the cytokine production assay, cells (5 × 10 6 ml −1 ) were stimulated for 12 h with ultrapure LPS (10 ng ml −1 ), Pam3CSK4 (100 ng ml −1 ), oxidized-zymosan (100 μg ml −1 ), DNFB (100 μg ml −1 ), oxazolone (10 μg ml −1 ), FITC (5 μg ml −1 ), BA (10 μg ml −1 ), MS (10 μg ml −1 ) or SLS (5 μg ml −1 ). Poly (dA:dT) (2 μg ml −1 ) was used as previously described [68] . For stimulation with ATP or silica for IL-1α and IL-1β production assay, cells were primed with 1 ng ml −1 ultrapure LPS for 3 h and then stimulated with ATP (5 mM) or silica (100 μg ml −1 ). For determination of intracellular pro-IL-1α and pro-IL-1β by ELISA, cells were stimulated in the presence of the pan-caspase inhibitor Z-VAD-fmk (100 μM) for 12 h and then lysed by repeated freeze–thaw cycling in PBS supplemented with a protease inhibitor cocktail (Complete mini, Roche). For treatment with chemical inhibitors, cells were preincubated with the lysosomal acidification inhibitor bafilomycin A (100 nM), the Syk inhibitor BAY61-3606 (3 μM), the P2X 7 inhibitor KN-62 (10 μM), the ATP-dependent potassium-channel inhibitor Glibenclamide (25 μM) or the ROS inhibitors APDC (50 μM) or NAC (10 μM) for 1 h before the addition of inflammasome activators. The culture supernatants or cell lysates were analysed using ELISA kits for TNF, IL-6, IL-12p70, IL-1α and IL-1β. For analysis of the phenotypic maturation of BMDCs, BMDCs were stimulated with TNBS (100 μg ml −1 ) for 24 h, stained with antibodies for CCR7, I-A b , CD80, CD86 and CD40, and analysed by flow cytometry using a MACSQuant Analyzer (Miltenyi Biotech) with gating on CD11c + PI − cells. Assay for ROS production BMDCs were treated with the indicated stimulants for 15 min at 37 °C, then mixed with 1 μM CM-H 2 DCFDA or 1 μM CellROX Deep Red Dye (only for FITC stimulation) and further incubated for 30 min at 37 °C. The cells were stained with anti-mouse CD11c APC and PI and analysed for fluorescence signals in CD11c + PI − cells by flow cytometry using a MACSQuant Analyzer (Miltenyi Biotech). Assay for caspase-1 activity Intracellular caspase-1 activity was detected using FLICA reagents (Immunochemistry Technologies) according to the manufacturer’s instructions. In brief, BMDCs were incubated for 8 h with the indicated stimulants in low-serum medium (RPMI1640 supplemented with 2% FBS). FAM-YVAD-fmk or 660-YVAD-fmk (only for FITC stimulation) were reconstituted in dimethyl sulfoxide and diluted 1:5 in PBS to prepare a working solution. The stimulated BMDC suspensions (10 4 cells per ml) and the FLICA working solution were mixed in a ratio of 50:1 and incubated for 60 min at 37 °C, followed by staining with anti-mouse CD11c APC (1:100) and PI, and then analysed for fluorescence signals within CD11c + PI − cells by flow cytometry using a MACSQuant Analyzer (Miltenyi Biotech). Re-stimulation of hapten-specific T cells ex vivo For in vitro re-stimulation of T cells from hapten-sensitized mice, auricular, maxillary and axillary lymph nodes were pooled, and a single-cell suspension was prepared. Thy1 + T cells (1 × 10 5 per well) purified using a MACS sorting system (Miltenyi Biotec) were co-cultured with irradiated (3,000 rad) TNP-modified syngeneic spleen cells (5 × 10 5 per well) as described, and concentrations of IL-17A and IFN-γ in the culture supernatants on day 3 were measured by ELISA. For preparation of T cells from Rag2 −/− mice reconstituted with T cells from WT mice congenic for Ly5.1 and MyD88 −/− or IL-1R1 −/− mice expressing Ly5.2, skin dLN cells were isolated 5 days after TNCB sensitization and sorted into Thy1.2 + Ly5.1 + (WT-derived) and Thy1.2 + Ly5.2 + ( MyD88 −/− or IL-1R1 −/− -derived) T cells by a FACS cell sorter (Aria II, BD). Sorted cells were re-stimulated with irradiated (3,000 rad) TNP-modified or unmodified syngeneic spleen cells, and the production of IL-17A and IFN-γ in the culture supernatants at day 3 was measured by ELISA. Immunoblot analysis For preparation of cell lysates of BMDCs, cells were stimulated at 37 °C for various periods of time with ox-zymosan (100 μg ml −1 ), TNBS (100 μg ml −1 ), oxazolone (10 μg ml −1 ), DNFB (100 μg ml −1 ), FITC (5 μg ml −1 ) or SLS (5 μg ml −1 ) and then lysed in ice-cold lysis buffer (50 mM Tris-HCl, pH 8.0, 150 mM NaCl, 1.0% Triton X-100, 20 mM EDTA, 1 mM Na 3 VO 4 , 1 mM NaF and protease inhibitor cocktail). For extraction of nuclear proteins from BMDCs, cells were stimulated for 90 min with LPS (10 ng ml −1 ), ox-zymosan (100 μg ml −1 ) or TNBS (100 μg ml −1 ), and then cells were suspended in ice-cold buffer A (10 mM HEPES [pH 7.8], 10 mM KCl, 0.1 mM EDTA, 1 mM DTT, 0.6% NP-40 and protease inhibitor cocktail). Nuclei were pelleted and suspended in ice-cold buffer C (20 mM HEPES [pH 7.8], 0.4 M NaCl, 1 mM EDTA, 1 mM DTT and protease inhibitor cocktail). After vortexing and stirring for 30 min at 4 °C, the samples were centrifuged, and the supernatants were collected. Cell lysates were separated by SDS–PAGE and proteins were transferred onto polyvinyldifluoride membranes (Amersham). Membranes were incubated with primary antibodies and then with horseradish peroxidase-conjugated secondary antibodies, followed by development with the ECL detection system (Amersham Pharmacia). Band intensities were quantified with a LAS-3000 imaging system (FUJIFILM). The Abs used were against Syk (1:1,000), p-Syk (Tyr525/526)(1:1,000), p-Syk (Tyr352) (1:1,000), NF-κB p65(1:500), c-Rel (1:500), α-tubulin (1:1,000) and lamin B (1:500). Statistical analyses An unpaired two-tailed Student’s t- test was used for all the statistical analyses. Differences with P- values <0.05 were considered significant. How to cite this article: Yasukawa, S. et al . An ITAM-Syk-CARD9 signalling axis triggers contact hypersensitivity by stimulating IL-1 production in dendritic cells. Nat. Commun. 5:3755 doi: 10.1038/ncomms4755 (2014).